Optimization of stress response through the nuclear receptor-mediated cortisol signalling network It is an accepted paradigm that extended stress predisposes an individual to pathophysiology. However, the biological adaptations to minimize this risk are poorly understood. Using a computational model based upon realistic kinetic parameters we are able to reproduce the interaction of the stress hormone cortisol with its two nuclear receptors, the high-affinity glucocorticoid receptor and the low-affinity pregnane X-receptor. We demonstrate that regulatory signals between these two nuclear receptors are necessary to optimize the body’s response to stress episodes, attenuating both the magnitude and duration of the biological response. In addition, we predict that the activation of pregnane X-receptor by multiple, low-affinity endobiotic ligands is necessary for the significant pregnane X-receptor-mediated transcriptional response observed following stress episodes. This integration allows responses mediated through both the high and low-affinity nuclear receptors, which we predict is an important strategy to minimize the risk of disease from chronic stress. There is a requirement for robustness within biological systems, defined as the ability of a system to undertake its core function despite external challenges [1] . Product inhibition, feed-forward and feed-back inhibition and stimulation, as well as repression and induction regulatory loops allow biological systems to approach both robustness and adaptability [2] . Biological systems are routinely exposed to external challenge, such as the stress response where each challenge causes a transient spike in blood cortisol, activating catecholamine production in the brain and glucose mobilization in the liver, forming the classical fight or flight response [3] . It is clear that prolonged or repeated stress is associated with the development of pathophysiology [4] , [5] , [6] ; for example, high stress police work is associated positively with the development of metabolic syndrome [7] , [8] . As such, it is both an important biological question, and challenging modelling scenario, to understand how these metabolic networks function efficiently, balancing both the pharmacodynamic (physiological effect of the challenge on the biological system) and pharmacokinetic (metabolic response to the challenge, leading to a return to homoeostasis) responses to stress: This ensures an efficient fight or flight response, while minimizing the overstimulation associated with increased morbidity. Many genes responsible for the body’s responses to chemical and environmental challenge are regulated by members of the nuclear receptor superfamily [9] . These ligand-activated transcription factors may be divided into receptors with high-affinity ligands ( K d ~nM; for example, the glucocorticoid receptor (GR)), and those with low-affinity ligands ( K d ~μM; for example, the pregnane X-receptor (PXR)) [9] , [10] . Regulatory signals have been identified between nuclear receptors, although the impact of these on target gene expression is at present equivocal. Examples of such regulation include the positive regulation of PXR by GR [11] ; the positive regulation of PXR by peroxisome proliferator activated receptor α [12] , and the negative autoregulation of GR, progesterone receptor, androgen receptor and PXR on their own expression [13] , [14] , [15] . Indeed, the nuclear receptor network in its entirety holds multiple interlinked complex regulatory mechanisms [16] , [17] , the quantitative importance of which is only just becoming clear. Using a systems biology approach we reproduce a portion of this regulatory network in silico , based on both literature and on de novo -generated data, and demonstrate that the model can reproduce the known interactions between glucocorticoids, their cognate receptors and target gene sets. We demonstrate the utility of feed-forward and feed-back regulatory signals in optimizing the response to a stress challenge. Importantly, we demonstrate that the regulatory network only functions as a direct result of the promiscuity of the PXR ligand profile, with integration from multiple, low-affinity endogenous chemicals being obligate for activation of PXR by the nanomolar concentrations of cortisol released during a stress response. Finally, as multiple stress exposures are a more likely scenario in the real world, we examine how the system responds to repeated stimuli of differing frequency. We demonstrate that the network is robust towards low frequency perturbations, shows adaptation at moderate stress frequencies, but transitions to an altered steady state at high frequency stimulation, which we predict is predisposing towards stress-induced pathologies. Model generation and validation We generated an in silico model of the regulatory signal network known to regulate body responses to glucocorticoids in the human liver, allowing examination of both pharmacodynamic and pharmacokinetic responses to stress. 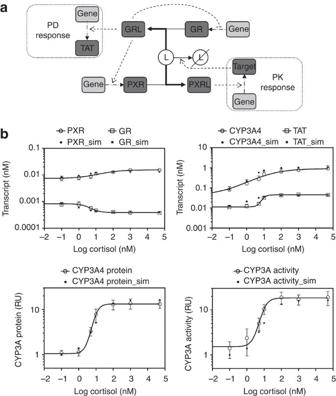Figure 1: Regulatory signal network under study and model validation. (a) A single ligand (L) acts as an agonist for both PXR and GR, forming an activated complex (hashed outline). Activated GR controls both the expression of target genes involved in the pharmacodynamic effect cortisol (for example, the expression of TAT) of its ligand L (often cortisol) and PXR expression. Activated PXR controls the expression of target gene involved in the pharmacokinetic response (for example, CYP3A4), which acts to remove the stimulating ligand (L). (b) Primary human hepatocytes were exposed to vehicle or (0.1–50000, nM) cortisol as indicated for 48 h, RNA extracted and transcript levels of PXR, GR, CYP3A4 and TAT quantified by TaqMan quantitative PCR. Average transcript levels (±s.e.m.) from triplicate cultures are indicated by open symbols, and the concentration-response curve shown by the full line was fitted to these data. Transcript levels of PXR, GR, CYP3A4 and TAT following 48 h exposure to indicated concentrations of cortisol were also simulated by the model, and are presented as closed symbols. (c) Primary human hepatocytes were as above and total protein extracted. CYP3A4 protein and activity levels were measured, with the average (±s.e.m.) from triplicate cultures indicated by open symbols, with concentration-response curve again fitted to the experimental data. Simulations of CYP3A4 protein and activity levels are presented as closed symbols. Figure 1a represents a cartoon of the basic network structure, while Supplementary Fig. S1 provides the complete model in Systems Biology Graphical Notation format and Supplementary Tables S1–S4 the model parameters, balance equations, conserved moieties and initial conditions used to populate the model, respectively. Within this model, cortisol (ligand ‘L’) may interact with two nuclear receptors; the high-affinity GR and the low-affinity PXR. Activation of GR by ligand, forming the GR-ligand complex (GRL), has three effects on the network: First, a feed-back regulatory signal causes transcriptional repression of GR [13] ; second, a feed-forward regulatory signal increases PXR expression, again at the transcriptional level [11] ; third, GRL upregulates the transcription of a target gene set, including the classic marker gene tyrosine aminotransferase (TAT [18] ), which we use to represent the pharmacodynamic response. Activation of PXR by ligand (forming PXRL) has a single action; stimulation of a second target gene set, including the marker gene CYP3A4 (ref. 19 ). The reduction in concentration of ligand L by an enhanced activity of CYP3A4 is incorporated into the model, allowing us to simulate the dynamic response to ligand challenge, and making CYP3A4 a surrogate marker for the pharmacokinetic response. It should be noted that while heterologous overexpression experiments have shown that GR activation can have an impact on CYP3A4 reporter gene expression [20] other in vitro experiments clearly demonstrate that any interaction must be indirect as there is no consensus GR response element within the CYP3A4 regulatory region [21] , and GR ChIP-Seq experiments fail to demonstrate a direct interaction [22] , [23] . Figure 1: Regulatory signal network under study and model validation. ( a ) A single ligand (L) acts as an agonist for both PXR and GR, forming an activated complex (hashed outline). Activated GR controls both the expression of target genes involved in the pharmacodynamic effect cortisol (for example, the expression of TAT) of its ligand L (often cortisol) and PXR expression. Activated PXR controls the expression of target gene involved in the pharmacokinetic response (for example, CYP3A4), which acts to remove the stimulating ligand (L). ( b ) Primary human hepatocytes were exposed to vehicle or (0.1–50000, nM) cortisol as indicated for 48 h, RNA extracted and transcript levels of PXR, GR, CYP3A4 and TAT quantified by TaqMan quantitative PCR. Average transcript levels (±s.e.m.) from triplicate cultures are indicated by open symbols, and the concentration-response curve shown by the full line was fitted to these data. Transcript levels of PXR, GR, CYP3A4 and TAT following 48 h exposure to indicated concentrations of cortisol were also simulated by the model, and are presented as closed symbols. ( c ) Primary human hepatocytes were as above and total protein extracted. CYP3A4 protein and activity levels were measured, with the average (±s.e.m.) from triplicate cultures indicated by open symbols, with concentration-response curve again fitted to the experimental data. Simulations of CYP3A4 protein and activity levels are presented as closed symbols. Full size image The model is defined by series of balance and rate equations. Where available, parameters were taken from the literature ( Supplementary Table S1 ), with the remaining parameters fitted to the known biological behaviour of the system, while maintaining these parameters within biologically realistic bounds (for example, average gene transcription rate). Using these specifications, the model corresponds to the most realistic possible considering the current state of knowledge. The model was validated by reproducing the response of primary human hepatocytes exposed to the glucocorticoid cortisol. Cortisol is a high-affinity GR ligand ( K d =10 nM, [24] ), and a low-affinity PXR ligand ( K d =10 μM, ref. 24 ). As can be seen from Fig. 1b , the model replicates the dose-dependent modulation of GR, PXR, CYP3A4 and TAT steady-state mRNA levels observed in primary human hepatocytes exposed to cortisol; moreover, the model was able to qualitatively replicate the increases in CYP3A4 protein and activity levels observed in primary human hepatocytes ( Fig. 1c ). Furthermore, the model replicates the effect of the artificial glucocorticoid dexamethasone on primary human hepatocytes ( Supplementary Fig. S2 ). All the predicted changes were half complete at cortisol concentrations of ~10 nM, equivalent to the K d for its binding to GR. This is readily understood for TAT, GR and PXR as they are all impacted by the level of GRL. CYP3A4 mRNA and protein concentrations were also half regulated at 10 nM cortisol, which is potentially counterintuitive as CYP3A4 expression is regulated by PXRL, and yet the K d between cortisol and PXR is ~1,000-fold higher than this. As such, the need for further examination of the network is clear. These results demonstrate that the generated in silico network was sufficiently parameterized to allow meaningful interrogation of the biological scenario. It should be noted that although these data prove the model competent to describe the variations in the indicated species following cortisol challenge, they do not conclusively prove the fidelity of the model for other properties and perturbations. Impact of GR-mediated feed-back regulatory signal on network GRL invokes both a negative feed-back loop on GR expression and a positive feed-forward regulation on PXR transcription. To examine the importance of these regulatory interactions, we simulated the dynamics of the network following a sustained increase of cortisol levels. We then determined the importance of the two regulatory interactions by disabling either the negative feed-back loop (a network variant we shall refer to as ‘GRstubborn’), or the positive feed-forward regulation (the ‘PXRstubborn’ variant). In the wild-type network, a decrease in both the transcript and protein levels of GR were simulated in response to a sustained intracellular level of 10 nM cortisol, confirming the operation of the GR-mediated autoregulatory feed-back loop ( Fig. 2a ). In addition, the increases in both PXR transcript and protein levels were semi-transient in nature, with the reduction of PXR expression by GRL via the feed-forward signal providing the mechanistic rationale. Simulation of the same exposure on the GR stubborn network predicted no alteration in transcript or protein levels for GR (both GR+GRL) and a persistent elevation in PXR due to the sustained higher GRL levels ( Fig. 2a ). Hence, the GR-mediated negative feed-back loop can be seen to impact upon levels of GR (directly) and PXR (indirectly). 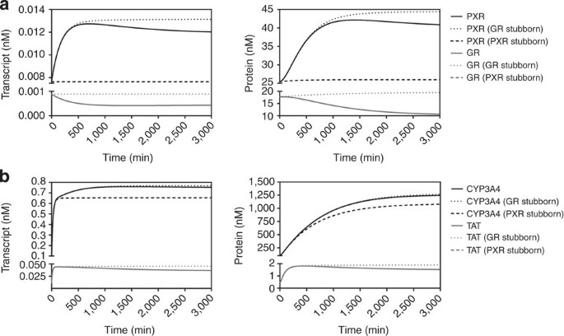Figure 2: GR-mediated negative feed-back on GR expression. Transcript and protein levels for (a) GR and PXR, and (b) CYP3A4 and TAT, were simulated over 3,000 min following addition (in silico) of cortisol to a constant level of 10 nM. Solid lines represent levels simulated for the complete single-ligand model, whereas dashed lines represent levels GR stubborn and PXR stubborn scenarios as indicated. Figure 2: GR-mediated negative feed-back on GR expression. Transcript and protein levels for ( a ) GR and PXR, and ( b ) CYP3A4 and TAT, were simulated over 3,000 min following addition ( in silico ) of cortisol to a constant level of 10 nM. Solid lines represent levels simulated for the complete single-ligand model, whereas dashed lines represent levels GR stubborn and PXR stubborn scenarios as indicated. Full size image The GR negative feed-back loop also impacts on the expression of GR and PXR target genes. The negative feed-back loop acts to attenuate expression of the classical GR target gene TAT ( Fig. 2b ), with the GR stubborn variant resulting in a predicted temporal persistence of TAT expression. This negative feed-back loop also produces a modest decrease in the long-term expression of the PXR target gene CYP3A4 ( Fig. 2b ). Impact of GR-mediated feed-forward regulatory signal We next examined the role of the GR-mediated feed-forward signal, whereby GRL stimulates PXR gene expression. The PXR stubborn variant predicted no alteration in transcript or protein levels for PXR, or TAT and GR in response to 10 nM intracellular cortisol, the latter being understandable as their regulation is controlled upstream of this regulatory loop within the network ( Fig. 2a ). For the PXR stubborn variant, the increase in CYP3A4 levels following 10 nM intracellular cortisol was less than simulated in the complete model, but the change in Area Under the concentration-time Curve (AUC) was modest (~15%: Fig. 2b ). The molecular rationale behind this apparent lack of control becomes clear if the relative affinities of cortisol towards PXR and GR are considered: The K d of cortisol for PXR is ~1,000-fold higher than the K d for GR. A biologically realistic maximal intracellular concentration for cortisol is 10 nM, as used in this simulation, and results in 50% occupancy of GR ( K d ≈10 nM), but only 0.1% occupancy for PXR ( K d ≈10 μM). Under the simulated exposure paradigm, total PXR protein level is predicted to increase by 17 nM due to the GRL-mediated feed-forward regulatory signal. However, this results in an increase of PXRL of <0.02 nM, producing a very small impact on PXR target gene expression. Given that these conditions are biologically realistic with respect to receptor and ligand concentrations, plus the affinity of cortisol for both GR and PXR, we are left with a paradox; why does a feed-forward regulatory signal exist that appears poorly functional under normal biological conditions? To answer this apparent paradox, we further considered the basic biology of PXR. Although originally described as a promiscuous nuclear receptor with many endogenous and xenobiotic ligands [26] , [27] , [28] , PXR has largely become thought of as a xenosensor [29] , [30] . Recent work has refocused on the role of PXR in endogenous processes [15] , [31] , [32] , and we would suggest that the known feed-forward regulation of PXR expression by endosensing steroid hormone receptors such as the GR, ER and PPAR [11] , [14] would be supportive of such a role. At any given time the intracellular milieu will contain a number of low-affinity endogenous PXR ligands, and we must, therefore, consider not only the role of individual endobiotic ligands, but also their collective effect. Each of these ligands (L 1 …L n ) individually is present in the cell at a low concentration (nM), and coupled with low affinities ( K d ≈μM) occupancy of PXR by any one ligand (PXRL 1 ...PXRL n ) would be negligible. However, if the levels of these endogenous ligands are integrated, then it should be possible to achieve a total ligand pool that will result in a significant level of PXR occupancy. This would result in a higher level of activated PXR under baseline conditions, and hence PXR target genes such as CYP3A4. Importantly, the GR-mediated feed-forward regulatory signal means that cortisol challenge now has an unexpected effect; increased PXR leads to not only an increase in PXRL (for example, PXR activated by cortisol) but also PXRL 2 ..PXRL n (for example, PXR activated by all other endogenous ligands, hereafter referred to as ligand pool L2). To examine this scenario we introduced a second ligand pool (L2), representing the integration of all endogenous ligands for PXR present within the cell. This pool was set to a concentration of 100 nM, with a K d =10 μM, which we believe is not inconsistent with a biologically realistic value. The model parameters, balance equations, conserved moieties and initial conditions used to populate this model are presented in Supplementary Tables S5–S8 , respectively. Following addition of the second ligand pool, the impact of cortisol challenge to a sustained intracellular level of 10 nM on the network was simulated for the wild-type, GR stubborn and PXR stubborn networks ( Fig. 3 ). As predicted, the presence of the L2 ligand pool had little impact upon the dynamic response of PXR, GR or TAT. For CYP3A4, however, two notable effects were predicted: First, the transcript and protein levels were significantly higher under the steady-state baseline before cortisol addition (1,628 nM versus 111 nM for L1+L2 and L1 alone, respectively). Second, the GR-mediated feed-forward regulatory signal is now fully functional, being responsible for ~80% of the increase in CYP3A4 AUC observed upon cortisol challenge. This strong dependence on the feed-forward regulation is understandable as added cortisol has a dual effect on CYP3A4 expression; the first is rapid and due to binding of L to pre-existing PXR. The second is slower and is due to binding of L and L2 to PXR that is produced de novo through the action of the GRL-mediated feed-forward regulatory signal. Together, these effects increase the total activated PXR pool (PXRL+PXRL2) by over 10-fold compared with PXRL alone. 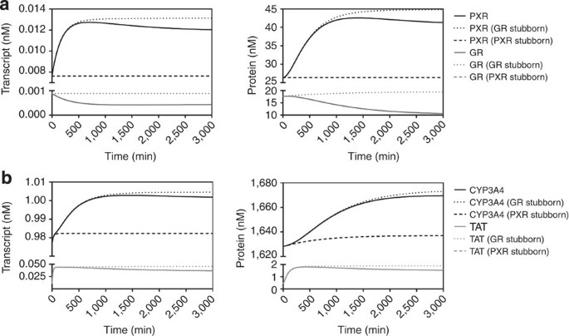Figure 3: Integration of endogenous ligand concentrations by PXR. Transcript and protein levels for (a) GR and PXR, and (b) CYP3A4 and TAT, were simulated over 3,000 min following addition (in silico) of cortisol to a constant level of 10 nM. In all simulations, an additional PXR ligand pool (L2) of concentrations equal to 100 nM was present. Solid lines represent levels simulated for the complete single-ligand model, whereas dashed lines represent levels GR stubborn and PXR stubborn scenarios as indicated. Figure 3: Integration of endogenous ligand concentrations by PXR. Transcript and protein levels for ( a ) GR and PXR, and ( b ) CYP3A4 and TAT, were simulated over 3,000 min following addition (in silico) of cortisol to a constant level of 10 nM. In all simulations, an additional PXR ligand pool (L2) of concentrations equal to 100 nM was present. Solid lines represent levels simulated for the complete single-ligand model, whereas dashed lines represent levels GR stubborn and PXR stubborn scenarios as indicated. Full size image An intriguing extension of this prediction is that L2 ligand pool size actually drives target gene induction, with larger L2 pools producing significantly more activated PXR (PXRL+PXRL2) due to the GR-mediated feed-forward regulatory signal. Supplementary Fig. S3 demonstrates that as L2 pool size increases, so does the predicted basal expression of CYP3A4, while the degree to which it can be further induced decreases. This inverse correlation is supported by literature data, where fold induction of metabolic enzymes in primary human hepatocytes was observed to be inversely correlated with their basal expression level for a range of inducers [33] . Dynamics of the network following multiple stress episodes All previous simulations were undertaken using a fixed intracellular concentration of 10 nM cortisol, consistent with our experimental model system. However, a more clinically relevant scenario involves an acute spike of cortisol released into the bloodstream following a stress episode. Moreover, in modern society many individuals are exposed to a number of stress events sequentially. We thus used the complete model to ask how the gene regulatory network responds to repeat blood cortisol spikes, equivalent to sequential stress episodes. Three different frequencies of stress episodes were examined; 1 per week, 1 per day or 1 per hour, corresponding to ‘low-’, ‘medium-’ and ‘high-’ stress scenarios. Simulated protein levels for each of these scenarios are presented in Fig. 4 , with transcript level simulations as Supplementary Data ( Supplementary Fig. S4 ). In the low-stress scenario all species were predicted to return to baseline following each stress episode, making each stress response independent. In contrast, the medium stress scenario produces new mean expression levels for all species, with protein levels oscillating around this new mean. For TAT, this mean approximates the maximal level of TAT expression seen during the low-stress scenario; in contrast, GR, PXR and CYP3A4 variances are greater. These data are consistent with an adaptive response, where the network has moved to a new steady state that acts to limit the magnitude of the pharmacodynamic response, as measured by TAT expression. It is of particular note that while there is a substantial increase in blood cortisol between low and moderate frequency scenarios (AUC=fivefold increase and C max=2.9-fold increase), the increase in TAT levels is significantly less (AUC=3.6-fold increase and C max=1.6-fold increase): This is consistent with a successful adaptation to medium frequency stress. However, high stress conditions predict large variances in all species in the model, suggesting a failure to adapt. We suggest that the resultant permanent increase in pharmacodynamic response, as measured by TAT expression, represents overstimulation and a predisposition to increased morbidity. It is also important to note that alteration in non-GR target genes may be important in modulating morbidity. For example, expression levels of the PXR target gene CYP3A4, are predicted to increase dramatically in the high stress scenario (AUC=12.8-fold increase and C max=9.2-fold increase), and as CYP3A4 is responsible for the metabolism of a large number of endogenous steroids [19] , [30] this may impact upon the homoeostasis of these steroids, also contributing to increased morbidity. Despite this failure to adapt, the network can still minimize the impact of high stress to some degree; a dramatic increase in blood cortisol levels compared with the low-stress scenario is observed (AUC=89-fold increase and C max=31.4-fold increase), but the increase in TAT expression levels is significantly muted (AUC=7-fold increase and C max=2.4-fold increase). 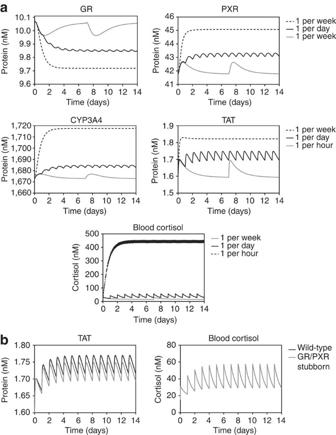Figure 4: Response of the gene regulatory network to repeat stress episodes. (a) Protein levels for GR, PXR, CYP3A4 and TAT, as well as free blood cortisol, were simulated over 21 days following addition of repeat spikes of cortisol, such that each spike doubled the free blood cortisol concentration. Frequency of cortisol spikes were 1 per week (grey line), 1 per day (black line) or 1 per hour (dashed line). (b) TAT and free blood cortisol were simulated as above, but under wild-type (black line) and GR/PXR stubborn (grey line) network variants. Figure 4: Response of the gene regulatory network to repeat stress episodes. ( a ) Protein levels for GR, PXR, CYP3A4 and TAT, as well as free blood cortisol, were simulated over 21 days following addition of repeat spikes of cortisol, such that each spike doubled the free blood cortisol concentration. Frequency of cortisol spikes were 1 per week (grey line), 1 per day (black line) or 1 per hour (dashed line). ( b ) TAT and free blood cortisol were simulated as above, but under wild-type (black line) and GR/PXR stubborn (grey line) network variants. Full size image Finally, we simulated the TAT and blood cortisol levels under conditions of moderate frequency stress episodes, for both the wild-type network and a variant where both GR-mediated regulatory signals had been disabled (GR/PXR Stubborn variant). The regulatory signals have no impact on the blood cortisol level, but the level of TAT was significantly impacted by the GR/PXR stubborn variant, with 1.3-fold increases in both AUC and Cmax compared with the wild-type network simulated ( Fig. 4 ). From this we can conclude that the main action of the regulatory signals is to minimize the pharmacodynamic response to repeated stress episodes, effectively de-sensitizing the body to chronic stress. Adaptation to chronic stress is re-enforced through low-stress periods One of the design features of the network simulated herein is the ability to adapt to moderate levels of stress. Given that workdays are, generally, more stressful than non-workdays, we asked if a weekend break was beneficial for our ability to respond to moderate stress, and if an extended vacation was even better. 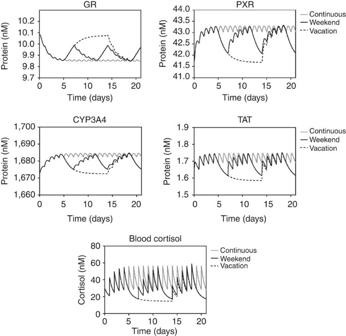Figure 5: A low-stress vacation is required to allow adaptation to a stressful week. Protein levels for GR, PXR, CYP3A4 and TAT, as well as free blood cortisol, were simulated over 21 days following addition of repeat spikes of cortisol, such that each spike doubled the free blood cortisol concentration. Cortisol spikes were applied 1 per day for either continuous throughout the period (grey line), with a weekend break (black line) or a 9-day vacation (dashed line). Figure 5 shows the simulated protein levels of all species following once per day stress events under three scenarios: continuous stress every day for 21 days; a weekend scenario with 5 days of stress, followed by 2 days with no stress, for 21 days; a vacation scenario with 5 days of stress, followed by 9 days with no stress, and then 5 days of stress. Transcript levels are presented in Supplementary Fig. S5 . In the weekend scenario, predicted levels mirrored the 21-day constant stress scenario for the first 5 days, as expected. Protein levels for all species were predicted to return towards baseline during the low-stress weekend, but did not fully recover. TAT protein levels were predicted to reach 82% of their baseline value, while PXR and CYP3A4 reached 75% and 77%, respectively. In contrast, GR protein levels were predicted to only reach 45% of their baseline value. The net effect of this is a ‘biological memory’ within the network to the first stress episode. However, the impact of this biological memory is, perhaps surprisingly, minimal, with the response to stress on day 8 being only negligibly smaller than on day 1. However, during a 9-day vacation there appears to a significant memory effect, with the response to stress on the first day back from vacation being significantly less that the response seen on day 1. Figure 5: A low-stress vacation is required to allow adaptation to a stressful week. Protein levels for GR, PXR, CYP3A4 and TAT, as well as free blood cortisol, were simulated over 21 days following addition of repeat spikes of cortisol, such that each spike doubled the free blood cortisol concentration. Cortisol spikes were applied 1 per day for either continuous throughout the period (grey line), with a weekend break (black line) or a 9-day vacation (dashed line). Full size image The glucocorticoid class of steroid hormones undertake a large number of functions central to normophysiology; additionally, they respond to external stress challenge, producing the ‘fight or flight’ response [34] . Much recent interest has focussed on the association between chronic stress and predisposition towards disease states, including a number of complex pathologies such as metabolic syndrome [4] , [35] , hippocampal vulnerability [6] , depression [36] and drug–induced liver injury [37] . Using a systems modelling approach we have examined the regulatory signal network that underlies the cortisol-driven stress response under both normophysiology and following stress episodes. The signal regulatory network is centred around the interaction of the stress hormone cortisol with two nuclear receptors; a high-affinity ligand with GR, and low-affinity ligand with PXR (~1,000-fold difference in K d ). Glucocorticoids have previously been shown to activate feed-back and feed-forward regulatory signals on GR and PXR expression, respectively [11] , [13] , which we demonstrate are important in regulating the network response as a whole. As such, we describe an important emergent feature of the network; the buffering of TAT levels relative to cortisol level following repeat stress episodes, consistent with an adaptation to minimize the physiological response and reducthe risk of disease progression. Such data is consistent with the clinical observation of Kirschbaum et al. [38] , who examined the response of healthy men to daily stress events. In these individuals they observed that subsequent stress events causing a reduced response. Even under the high stress scenario, a large degree of buffering occurs; however, given the available human data we would suggest that this is insufficient to prevent a marked increase in morbidity. For example, the chronic stress associated with combat scenarios has been associated with generalized disease phenotypes, such as post-traumatic stress disorder [39] . In general, workdays are more stressful compared with weekends, yet our simulations predict that there is negligible difference between a stress response on day 1 of the medium stress scenario, and on day 8, following a weekend of no stress. In contrast, following a short vacation, we predict a muted response compared with the day 1 (naive) response. A potential explanation for this is the differential kinetics of cortisol and the GR: cortisol is degraded relatively quickly as CYP3A4 levels are high at the start of the vacation and remain so until the cortisol level drops sufficiently for the GRL-mediated feed-forward regulatory signal to become inactive and for PXR protein to then degrade. In contrast, GR levels are influenced by the level of GRL, which is auto-inhibitory on GR transcription. As such, the increase in GR expression level following cessation of the stress episodes is predicted to lag behind the decrease in cortisol levels as it is dependent upon both the initial loss of cortisol to terminate the GRL-mediated auto-inhibitory signal, and the need to transcribe and translate GR de novo . Whilst the impact of this differential kinetics cannot be seen following a short weekend break, over a 9-day vacation there is sufficient time for a positive memory to emerge, effectively de-sensitizing the network to further stress episodes. It should be noted that the model presented represents only a single portion of the entire biological system. We cannot exclude the possibility of compensatory changes to other proteins outside the modelled network. It would be expected that, for example, an increase in CYP3A4 levels would increase metabolism of its many endogenous substrates, initiating feed-forward regulatory signals to increase steroid synthesis and return to homoeostasis. Indeed, one potential reason for the evolution of such a regulatory signal network may be energy conservation, whereby a tight regulation of degradative processes is necessary to prevent futile energy expenditure through unnecessary anabolic processes. In addition, we provide a solution to the paradox that endogenous chemicals are often ligands for both low-affinity and high-affinity receptors. As intracellular levels of these steroid hormones are generally several orders of magnitude lower than their K d for low-affinity receptors, this suggests the level of PXRL will always remain low, and effectively biologically silent. Building on the knowledge that PXR is a promiscuous receptor with multiple endogenous ligands [26] , [27] , [28] we demonstrate that integration of these individual ligands (PXRL 1 …PXRL n ) results in a significant increase of PXRL, increasing transcriptional activation of PXR target genes at baseline. Furthermore, through the use of the feed-forward regulatory loop, whereby GRL increases PXR protein levels, a single ligand (for example, cortisol) can have a biologically important impact on activated PXR, impacting upon both its own occupation of PXR (PXRL) and other PXR ligands (PXRL 2 …L n ; PXRL2). In summary, we present a systems modelling approach to understand the design principles underlying the biological response to stress. We demonstrate that this network is able to regulate both the magnitude and duration of the physiological response to a stress episode, which we believe is an important design feature to protect against increased morbidity due to chronic overstimulation. In addition, we demonstrate that this system is robust against repeated stress episodes, producing only small variations in the physiological response for large increases of blood free-cortisol. Finally, we suggest that the differential kinetics of species within the network mean that a sustained vacation leads to a ‘biological memory’, lessening the response to subsequent stress episodes. Primary cell culture Primary human hepatocytes were a kind gift of GlaxoSmithKline, and were seeded at 2.4 × 10 5 cells cm −2 in 25 cm 2 flasks and allowed to attach overnight. Cells were dosed daily with vehicle, cortisol or dexamethasone (Sigma-Aldrich, Poole, UK) at the indicated concentrations. Following 48 h of exposure, total RNA and protein was isolated from quadruplicate samples. Total RNA was isolated using the RNeasy Mini kit (Qiagen, Crawley, UK) and quantified using a Nanodrop Agilent 2100 Bioanalyser, while total protein was extracted in RIPA buffer (1 × PBS, 1% Nonidet P40, 0.5% sodium deoxycholate, 0.1% SDS, protease inhibitor cocktail). Transcript level measurement Primers and TAMRA/FAM dual-labelled probe specific for PXR, GR, CYP3A4 and 18S were designed using the Primer Express software (Applied Biosystems, Warrington, UK) and were purchased from Eurofins (Wolverhampton, UK). Total RNA was treated with RNase-free DNase (Promega, Southampton, UK) to remove genomic contamination. Reverse transcription was primed with random hexamers and carried out by Superscript II (Invitrogen) as per the manufacturer’s instructions. To ensure that DNase-treated samples were free from genomic contamination a reverse-transcriptase negative control (lacking enzyme) was carried out for every RNA sample. Complementary DNA generated from 50 ng (PXR, GR, TAT and CYP3A4) or 50 pg (18S rRNA) of total RNA was amplified using TaqMan Universal polymerase chain reaction (PCR) Master Mix with 400 nM primers and 200 nM fluorogenic probe in a total reaction volume of 25 μl. Quantitative PCR reactions were run on the ABI7000 SDS instrument and quantified out using the ABI proprietary software against a standard curve generated from human genomic DNA (Promega). Protein level measurement Total protein extracts (10 μg per lane) were resolved on 12% SDS-polyacrylamide gels and then transferred electrophoretically to Hybond ECL nitrocellulose membranes (Amersham Biosciences, Little Chalfont, Bucks, UK). Membranes were blocked (1 h) in 5% fat-free dried milk and then probed with primary antibodies against human PXR (SAB2101636, 1:350; Sigma-Aldrich) or α-actin (sc1616, 1:500; Autogen Bioclear), followed by anti-rabbit IgG (sc2030, 1:10000; Autogen Bioclear) or anti-goat IgG (sc 2020, 1:20,000; Autogen Bioclear), respectively. Bound antibodies were visualized using enhanced chemiluminescence reagents according to the manufactures instructions (Amersham Biosciences). CYP3A4 protein activity measurement CYP3A4 enzyme activity was determined using the P450-Glo activity system (Promega, Southampton, UK), as per the manufacturer’s instructions. Briefly, Luciferin-PPXE substrate was mixed with S9 protein extract from primary human hepatocytes, along with an nicotinamide adenine dinucleotide phosphate regeneration system and detection reagent. Following 20-min incubation, luminescence was quantified using a Packard Lumicount. In silico modelling In silico models were generated using CellDesigner (v4.0.1; Systems Biology Institute, http://celldesigner.org/index.html ), a graphical front-end for creating process diagrams of biochemical networks in systems Biology Markup Language (ref. 28 ). Each individual chemical or protein is identified as a species (s1.....sn), while interactions between species are identified as reactions (r1....rn). For each reaction, a kinetic term can be included, detailing the mathematics underlying the interaction between the species. For more complex analysis, CellDesigner-generated models were transferred to COPASI (v4.6, build 32) (ref. 40 ), which is another Systems Biology Markup Language-compliant programme, but with a wider variety of analysis options. A number of the parameter values used within the model were fitted to the known biological behaviour of the system, while maintaining these parameters within previously determined biologically realistic bounds. To examine the robustness of the conclusions drawn within this paper we undertook a sensitivity analysis for these eight parameters. As detailed in Supplementary Tables S9 and S10 , our conclusions were mostly robust for up to a 10-fold change in any individual parameter value. The only exception was the expression level of CYP3A4 within Fig. 3 , as affected by the rate of GRL-dependent PXR transcription; K d of PXRL to CYP3A4 gene; and the rate of PXRL-dependent CYP3A4 transcription. Given that sensitivity is only observed for Fig. 3 , where a second ligand pool is included, and not in Fig. 2 , where the L2 pool is absent, it is logical to conclude that the L2 pool is, at least in part, responsible for the observation. We conclude that the increased basal expression of CYP3A4 due to the L2 pool may decrease the robustness of the system to fluctuations in these parameters. Importantly, despite this altered behaviour, decreased levels of CYP3A4 are more pronounced in the PXR stubborn variant, which is consistent with the central conclusions of this paper. How to cite this article: Kolodkin, A. et al. Optimization of stress response through the nuclear receptor-mediated cortisol signalling networks. Nat. Commun. 4:1792 doi: 10.1038/ncomms2799 (2013).